Blurry topography for precise target-distance computations in the auditory cortex of echolocating bats Echolocating bats use the time from biosonar pulse emission to the arrival of echo (defined as echo delay) to calculate the space depth of targets. In the dorsal auditory cortex of several species, neurons that encode increasing echo delays are organized rostrocaudally in a topographic arrangement defined as chronotopy. Precise chronotopy could be important for precise target-distance computations. Here we show that in the cortex of three echolocating bat species ( Pteronotus quadridens , Pteronotus parnellii and Carollia perspicillata ), chronotopy is not precise but blurry. In all three species, neurons throughout the chronotopic map are driven by short echo delays that indicate the presence of close targets and the robustness of map organization depends on the parameter of the receptive field used to characterize neuronal tuning. The timing of cortical responses (latency and duration) provides a binding code that could be important for assembling acoustic scenes using echo delay information from objects with different space depths. Echolocating bats use the time elapsed from biosonar pulse emission to the arrival of echo (defined as echo delay) to infer target distance. In the auditory cortex, echo delay is encoded by delay-tuned neurons that respond to pulse–echo pairs presented at specific delays [1] , [2] , [3] . Cortical delay-tuned neurons of the species Pteronotus parnellii , Pteronotus quadridens , Carollia perspicillata and Rhinolophus rouxi are confined to a specialized region in the dorsal auditory cortex defined as the frequency-modulated (FM)/FM processing area [4] , [5] , [6] , [7] . Some empirical evidence suggests that the FM/FM area has a role in the bat’s perception of echo delay [8] . In the FM/FM area, neurons are organized topographically according to their delay tuning and form a target-distance map based on echo-delay information. Neurons tuned to short delays (and hence short target distances) are found rostrally, whereas neurons tuned to longer delays are located more caudally [3] , [5] , [6] , [7] , [9] . This organizational pattern was termed ‘chronotopic organization’ because it describes how time information (in the form of echo delay) is represented in the cortex [6] , [9] . It has been hypothesized that activation of specific loci in the chronotopic map is important for an accurate perception of target range [4] , [10] , [11] . Chronotopic maps constitute one of many examples of topographies found in the mammalian neocortex. A widely used approach for the study of cortical organization is to calculate tuning properties of neurons while taking into account their position along the cortical surface [12] , [13] , [14] , [15] , [16] , [17] . Measuring neuronal tuning represents a problem because receptive fields are multiparametric, that is, neurons are driven by several combinations of stimulus features. The multiparametric nature of receptive fields is a source of bias to cortical maps. This is seen in computational maps such as the map of sound-source location in the owl’s tectum in which the receptive field of adjacent neurons largely overlaps and, therefore, the map appears more coarse than precise [18] , [19] . Moreover, in structural maps such as the tonotopic/cochleotopic map in the cat and the mouse primary auditory cortex, a precise tonotopic arrangement of neurons is observed if tuning is calculated with near-threshold stimuli but not if tuning is calculated at suprathreshold levels [20] , [21] . The response of delay-tuned neurons of bats has been described as multiparametric. The spike output of a delay-tuned neuron can be modified by several parameters including echo delay, echo level, pulse level and call repetition rate, among others [2] , [3] . One approach that captures at least some of the multiparametric nature of receptive fields of delay-tuned neurons is to calculate delay response fields (DRFs). DRFs represent the spike output of a neuron in the two-dimensional (2D) space of echo delay and echo level ( Fig. 1 ) [2] , [3] , [7] , [22] . 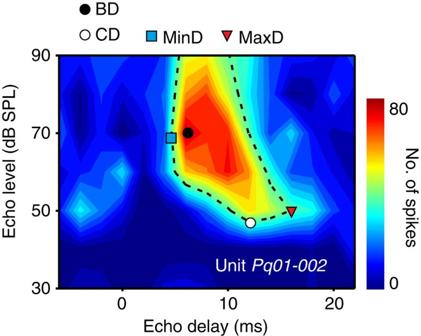Figure 1: The DRF of a neuron recorded inP. quadridens. The number of spikes in response to different combinations of echo delays and echo levels are colour coded. The dashed line indicates the threshold curve, calculated as 50% of the maximum response. Different parameters used for characterization of DRFs are indicated. BD, best delay; CD, characteristic delay; MaxD, maximum delay that was able to drive the neuron; MinD, minimum delay that was able to drive the neuron. Figure 1: The DRF of a neuron recorded in P. quadridens . The number of spikes in response to different combinations of echo delays and echo levels are colour coded. The dashed line indicates the threshold curve, calculated as 50% of the maximum response. Different parameters used for characterization of DRFs are indicated. BD, best delay; CD, characteristic delay; MaxD, maximum delay that was able to drive the neuron; MinD, minimum delay that was able to drive the neuron. Full size image The main purpose of this study was to explore the robustness of cortical target-distance representations by comparing target-distance maps obtained with different parameters that effectively characterize the DRFs. In other words, we wanted to know whether the multiparametric nature of delay-tuned responses obscures the cortical representation of the target distance of the bat. Our results show that the robustness of target-distance map organization depends on both the studied species and the parameter that is used for delay-tuning characterization. In the dorsal auditory cortex of three species of bats (that is, P. quadridens , P. parnellii and C. perspicillata ), the delay receptive field of adjacent neurons largely overlaps with most neurons responding to short target distances. We conclude that cortical target-distance representations are rather blurry than strictly and unequivocally ordered. Characteristics of DRFs DRFs were studied in the dorsal auditory cortex of three out of the four bat species in which the target-distance map have been demonstrated, precisely the sooty mustached bat ( P. quadridens ), the mustached bat ( P. parnellii ) and the short-tailed fruit bat ( C. perspicillata ). DRFs were obtained by measuring the neuronal response to changing echo delays and echo levels ( Fig. 1 ). Four parameters were used to describe receptive fields in the echo delay domain, precisely the echo delay of lowest threshold (defined as characteristic delay (CD)), the delay that produces the maximum number of spikes in the neuronal response (defined as best delay (BD)) and the minimum and maximum delays (MinD and MaxD, respectively) that were able to drive the neurons. The database used in this paper to study cortical topography is from the same units that were used in previous reports to describe basic aspects of delay tuning in the cortex of P. quadridens [7] , C. perspicillata [6] , [22] and P. parnellii [22] , [23] . Briefly, we gathered data from 12 adult P. quadridens , 10 adult P. parnellii and 9 adult C. perspicillata . A total of 119 delay-tuned neurons were recorded in the dorsal auditory cortex of P. quadridens , 89 neurons were recorded in P. parnellii and 111 neurons were recorded in C. perspicillata . In each species, 2D colour-coded histograms were calculated from the values of the different parameters used for characterization of DRFs and the level at which these measurements were taken ( Fig. 2 ). 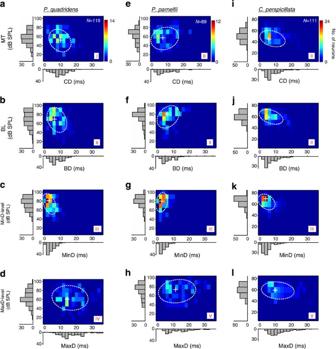Figure 2: Properties of DRFs. (a–d)P. quadridens, (e–h)P. parnellii, (i–l)C. perspicillata. (a,e,i) Distributions of CD and MT. (b,f,j) Distributions of BD and BL. (c,g,k) Distributions of MinD and the level at which it was measured (MinD level). (d,h,l) Distributions of MaxD and the level at which it was measured (MaxD level). Distributions are shown as one-dimensional and colour-coded 2D histograms. In the 2D histograms, the 75% error ellipsoids are given (dashed lines). The error ellipsoids were calculated from the covariance matrix of the 2D distribution and centred at the mean values. Plus (+) symbols indicate median values of each distribution. Roman numerals (white box inside the 2D histograms) indicate similarities and dissimilarities between 2D distributions. That there were differences in the 2D distributions of different parameters was checked with a factorial analysis of variance with multiple dependent variables (that is, delay value and echo-level value) and two categorical predictors (that is, species and type of DRF measure;P=0.0001,N=119 (P. quadridens),N=89 (P. parnellii),N=111 (C. perspicillata)). 2D histograms were grouped after apost-hoctest (Newman–Keuls method). Figure 2a,e,i show the 2D distribution of CD and the minimum threshold (MT) of each species. The CD–MT of a neuron indicates the echo delay and echo level to which a neuron is most sensitive. The CD–MT distribution calculated for P. quadridens was significantly different from that of P. parnellii and C. perspicillata ( Fig. 2a,e,i ). P. quadridens had more neurons that were maximally sensitive to echo delays close to 10 ms, whereas the other two species had more neurons that were maximally sensitive to shorter delays. Figure 2: Properties of DRFs. ( a – d ) P. quadridens , ( e – h ) P. parnellii , ( i – l ) C. perspicillata . ( a , e , i ) Distributions of CD and MT. ( b , f , j ) Distributions of BD and BL. ( c , g , k ) Distributions of MinD and the level at which it was measured (MinD level). ( d , h , l ) Distributions of MaxD and the level at which it was measured (MaxD level). Distributions are shown as one-dimensional and colour-coded 2D histograms. In the 2D histograms, the 75% error ellipsoids are given (dashed lines). The error ellipsoids were calculated from the covariance matrix of the 2D distribution and centred at the mean values. Plus (+) symbols indicate median values of each distribution. Roman numerals (white box inside the 2D histograms) indicate similarities and dissimilarities between 2D distributions. That there were differences in the 2D distributions of different parameters was checked with a factorial analysis of variance with multiple dependent variables (that is, delay value and echo-level value) and two categorical predictors (that is, species and type of DRF measure; P= 0.0001, N =119 ( P. quadridens ), N =89 ( P. parnellii ), N =111 ( C. perspicillata )). 2D histograms were grouped after a post-hoc test (Newman–Keuls method). Full size image The comparison of BD–best level (BL) distributions ( Fig. 2b,f,j ) did not reveal any apparent differences between species regarding target-distance sensitivity. The BL–BD of a neuron indicates the echo delay–echo level combination that produces the maximum number of spikes in the neuronal response. BD–BL histograms were similar across species and were also similar to the CD–MT histograms of P. parnellii and C. perspicillata . BD was positively correlated with the CD yielding correlation coefficients of 0.71 ( P. quadridens ), 0.83 ( P. parnellii ) and 0.91 ( C. perspicillata ; see Supplementary Fig. S1 ). The MinD-MinD level distributions also did not differ across species ( Fig. 2c,g,k ). The MinD of a neuron indicates the shortest echo delay that is able to reliably drive a neuron. The MinD–MinD level distributions were significantly different from CD–MT and BD–BL distributions both between and within species. The MinD–MinD level distributions were relatively sharp in the echo-delay domain. For example, the 75% error ellipsoids calculated in the 2D histograms had MinD borders between 0 and 6 ms ( P. quadridens and P. parnellii ), and between 0 and 9 ms ( C. perspicillata ). MinD was correlated with the CD yielding correlation coefficients of 0.62 ( P. quadridens ), 0.73 ( P. parnellii ) and 0.85 ( C. perspicillata ; see Supplementary Fig. S1 ). MaxDs and the levels at which they were obtained (defined as the MaxD level) indicate the longest echo delay that is able to drive a delay-tuned neuron. The MaxD–MaxD level distribution of P. quadridens significantly differed from that of P. parnellii and C. perspicillata ( Fig. 2d,h,l ). Remarkably, the MaxD–MaxD level histograms of all three species were quite broad, in particular when compared with the MinD–MinD level histograms. For example, the MaxD–MaxD level error ellipsoids covered MaxD ranges between 4 and 27 ms ( P. quadridens ), 1 and 24 ( P. parnellii ), and 1 and 21 ms ( C. perspicillata ). These MaxD ranges represent almost three times the range of echo delays contained in the MinD–MinD level error ellipsoids. In each species, the MaxD measure yielded the best correlation with the CD, that is, the CD–MaxD correlation coefficient had values of 0.74 ( P. quadridens ) and 0.92 ( P. parnellii and C. perspicillata ; see Supplementary Fig. S1 ). Cortical maps calculated with different DRF parameters Topographic organization of units according to the different DRF parameters was studied by pooling data from 12 adult P. quadridens , 10 adult P. parnellii and 9 adult C. perspicillata . The CD, BD, MinD and MaxD maps described in the succeeding text refer to the same cortical map (that is, the target-distance map) as visualized by different measures of delay tuning. Maps were constructed from the coordinates of each neuron relative to anatomic or functional landmarks (see Fig. 3 and Methods section) and colour coded for the value of the delay parameter that was being plotted. 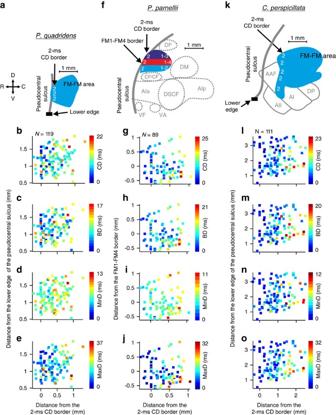Figure 3: Topographic organization of delay-tuned neurons. (a–e)P. quadridens, (f–j)P. parnellii, (k–o)C. perspicillata.(a,f,k) Position of the FM/FM area in relation to the pseudocentral sulcus (represented with thick grey lines). ForP. parnelliiandC. perspicillata, the positions of other auditory cortical areas are indicated. Reference points used for constructing composite maps are also indicated. In all three species, the 2-ms CD border was used as zero coordinate in the rostrocaudal axis. InP. quadridensandC. perspicillata, the lower edge of the pseudocentral sulcus was used as zero coordinate in the dorsoventral axis. InP. parnellii, the dorsoventral zero was set at the most ventral border of the FM1–FM4 stripe. The FM1–FM4 stripe was defined as the cortical region containing delay-tuned neurons that responded strongly to the echo delay between the fundamental (FM1) and the 4th biosonar harmonic (FM4), but that did not respond (or responded less) to other harmonic combinations (that is, FM1/FM2 or FM1/FM3). (b,g,l) Topographic organization of units according to CD. (c,h,m) Topographic organization according to BD. (d,i,n) Topographic organization according to the MinD. (e,j,o) Topographic organization according to the MaxD. In each species, the number of studied neurons is indicated in the CD maps. Figure 3: Topographic organization of delay-tuned neurons. ( a – e ) P. quadridens , ( f – j ) P. parnellii , ( k – o ) C. perspicillata. ( a , f , k ) Position of the FM/FM area in relation to the pseudocentral sulcus (represented with thick grey lines). For P. parnellii and C. perspicillata , the positions of other auditory cortical areas are indicated. Reference points used for constructing composite maps are also indicated. In all three species, the 2-ms CD border was used as zero coordinate in the rostrocaudal axis. In P. quadridens and C. perspicillata , the lower edge of the pseudocentral sulcus was used as zero coordinate in the dorsoventral axis. In P. parnellii , the dorsoventral zero was set at the most ventral border of the FM1–FM4 stripe. The FM1–FM4 stripe was defined as the cortical region containing delay-tuned neurons that responded strongly to the echo delay between the fundamental (FM1) and the 4th biosonar harmonic (FM4), but that did not respond (or responded less) to other harmonic combinations (that is, FM1/FM2 or FM1/FM3). ( b , g , l ) Topographic organization of units according to CD. ( c , h , m ) Topographic organization according to BD. ( d , i , n ) Topographic organization according to the MinD. ( e , j , o ) Topographic organization according to the MaxD. In each species, the number of studied neurons is indicated in the CD maps. Full size image Overall, maps of different DRF parameters confirmed the existence of a chronotopic arrangement of neurons along the rostrocaudal line ( Fig. 3 ). For example, neurons processing shorter delays (that is, blue-filled symbols in the maps of Fig. 3 ) were located more rostrally than neurons processing longer echo delays (red-filled symbols). In spite of the general chronotopy, the mere visual inspection of the different maps revealed that the chronotopic arrangement could be more apparent or less apparent, depending on the parameter that was used to characterize neuronal tuning and the species. For example, mapping the CD (Fig. 3b,g,l) and the MaxD (Fig.3e,j,o) produced the best apparent chronotopy, whereas maps constructed using MinDs (Fig. 3d,i,n ) appeared more blurry, at least in the two Pteronotus ( Fig. 3d,i ). For a quantitative comparison of maps constructed using different delay measures, we calculated the angular direction of local vector gradients and accumulated these angular directions in the form of circular histograms ( Fig. 4 ). In the circular histograms, the mean angular direction ( α ) indicates the orientation of the chronotopic axis, whereas the mean vector magnitude ( L α, calculated as: L α =1−distribution_variance) measures the strength of chronotopic organization. In every map, ‘ α ’ had values close to 0 rad, thus confirming a chronotopic arrangement of neurons that was almost perpendicular to the pseudocentral sulcus. 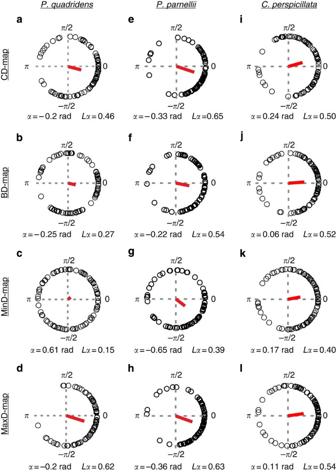Figure 4: Circular scatter plots characterizing the angular orientation of composite maps. (a–d)P. quadridens, (e–h)P. parnelliiand (i–l)C. perspicillata.Circular scatter plots were obtained by accumulating angle orientations of vector gradients calculated in individual animals. Open circles indicate angles of the gradient vectors. The red line points to the mean angular direction (α) of the circular distribution and its magnitude represents the mean vector magnitude (Lα, calculated as 1−variance). (a,e,i) Circular scatter plots calculated for CD maps. (b,f,j) Angle distributions calculated for BD maps. (c,g,k) Angle distributions calculated for MinD maps. (d,h,l) Angle distributions calculated for MaxD maps. The number of studied vector angles was 119, 111 and 89 forP. quadridens,P. parnelliiandC. perspicillata, respectively. Figure 4: Circular scatter plots characterizing the angular orientation of composite maps. ( a – d ) P. quadridens , ( e – h ) P. parnellii and ( i – l ) C. perspicillata. Circular scatter plots were obtained by accumulating angle orientations of vector gradients calculated in individual animals. Open circles indicate angles of the gradient vectors. The red line points to the mean angular direction ( α ) of the circular distribution and its magnitude represents the mean vector magnitude ( L α , calculated as 1−variance). ( a , e , i ) Circular scatter plots calculated for CD maps. ( b , f , j ) Angle distributions calculated for BD maps. ( c , g , k ) Angle distributions calculated for MinD maps. ( d , h , l ) Angle distributions calculated for MaxD maps. The number of studied vector angles was 119, 111 and 89 for P. quadridens , P. parnellii and C. perspicillata , respectively. Full size image As suspected from the visual inspection of maps, the level of organization along the rostrocaudal line varied depending on both the delay measure that was being studied and the species. Differences between maps constructed with different measures were more obvious in P. quadridens ( Fig. 4 ). In the CD and MaxD maps of P. quadridens , most gradient vectors were oriented between π /2 and − π /2; therefore, they pointed towards an increase of neuronal CD and MaxD in the rostrocaudal direction. In the CD and MaxD maps, L α had values of 0.46 and 0.62, respectively ( Fig. 4a,d ). On the other hand, vector angle distributions obtained from BD and MinD maps were more homogeneously organized around the circle (Rayleigh’s test, P= 0.06 (BD map) and P= 0.13 (MinD map); for both maps, the orientation of 119 vector gradients was analysed), therefore, yielding lower L α values, that is, 0.27 (BD map) and 0.15 (MinD map). In P. parnellii and C. perspicillata , there were no significant differences between vector angle distributions generated with all four studied delay measures (tested with a multisample test for equal median directions, P= 0.2 ( P. parnellii , 89 orientation vectors) and P= 0.72 ( C. perspicillata , 111 orientation vectors)). However, again the map of MinD was the one that was least organized in each species. For example, in P. parnellii and C. perspicillata the maps of CD, BD and MaxD yielded L α values above or equal to 0.5, but in the MinD map L α dropped to 0.39 ( P. parnellii ) and 0.40 ( C. perspicillata ). Overall, C. perspicillata was the species with the most reliable map across delay measures, for example, the largest L α difference observed between maps of C. perspicillata was of 0.14 (between MaxD and MinD maps) versus L α differences of 0.26 in P. parnellii (that is, between CD and MinD maps) and 0.47 in P. quadridens (that is, between MaxD and MinD maps). To better understand why cortical maps of MinD appeared less organized than maps of CD and MaxD, we looked into the DRFs of individual neurons recorded at different rostrocaudal positions ( Fig. 5 ). The three neurons depicted in Fig. 5a–c were recorded in one P. quadridens (denoted as Pq03 ) at 0.01, 0.26 and 0.8 mm from the estimated 2-ms border of CD. As expected, CD increased with the rostrocaudal position of the neurons, that is, the neuron located more rostrally ( Fig. 5a ) had a CD of 4 ms, the one in the middle of the map ( Fig. 5b ) had a CD of 8 ms, whereas the one in the more caudal position ( Fig. 5c ) had a CD of 14 ms. MaxD increased even more abruptly from a value of 6.8 ms (most rostral neuron) to 25 ms (most caudal neuron). On the other hand, the MinD of the three neurons remained relatively constant (that is, between 0 and 2 ms) across rostrocaudal coordinates. Abrupt changes in MaxD and slow changes in MinD along the rostrocaudal axis were also evident in individual examples of P. parnellii ( Fig. 5d–f ) and C. perspicillata ( Fig. 5g–i ), and when the entire set of neurons from all three species was analysed (see Supplementary Fig. S2 ). 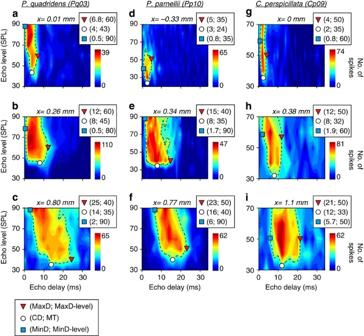Figure 5: DRFs of individual neurons recorded in different rostrocaudal positions. (a–c)P. quadridens, (d–f)P. parnelliiand (g–i)C. perspicillata.The example neurons ofP. quadridensandP. parnelliiresponded to FM1/FM2 harmonic combinations, whereas the example neuron ofC. perspicillataresponded to FM2/FM2 homohamormonic combinations. The rostrocaudal position of each neuron (relative to the 2-ms CD border) is given in the top of the DRF. In each DRF, the dashed line delineates the threshold curve of the neuron (calculated as 50% of the maximum activity in each DRF). The red triangle represents the MaxD of each neuron, the blue square represents the MinD and the open circle indicates the CD (see the square box at the bottom of the figure). The numbers besides each symbol give the value of the measured parameter (first number) and the level at which it was measured (second number). Figure 5: DRFs of individual neurons recorded in different rostrocaudal positions. ( a – c ) P. quadridens , ( d – f ) P. parnellii and ( g – i ) C. perspicillata. The example neurons of P. quadridens and P. parnellii responded to FM1/FM2 harmonic combinations, whereas the example neuron of C. perspicillata responded to FM2/FM2 homohamormonic combinations. The rostrocaudal position of each neuron (relative to the 2-ms CD border) is given in the top of the DRF. In each DRF, the dashed line delineates the threshold curve of the neuron (calculated as 50% of the maximum activity in each DRF). The red triangle represents the MaxD of each neuron, the blue square represents the MinD and the open circle indicates the CD (see the square box at the bottom of the figure). The numbers besides each symbol give the value of the measured parameter (first number) and the level at which it was measured (second number). Full size image Activation maps and population latencies In individual animals from all three studied species, activation maps were calculated to further explore the topographic aspect of chronotopic maps and the temporal characteristics of cortical activation. In the activation maps, the response of each neuron was treated as binary meaning that a neuron either responds or not to a given echo delay–echo level combination. A neuron was considered to respond to a given echo delay–echo level combination whenever it fired above 50% of the maximum response observed in the DRF. The criteria used here to define a response is the same as that used in previous studies to define the borders of DRFs [6] , [7] , [22] , [24] . Typical examples of activation maps of P. quadridens are shown in Fig. 6 . In the bat Pq02 , there was a clear chronotopic organization of units according to the CD ( Fig. 6a ). However, in response to echo delays below 10 ms and echo levels of 80 and 90 dB SPL, activation maps showed responses from units throughout the FM/FM area ( Fig. 6b ). Activation of units as expected from the chronotopic map (that is, only rostral units responding to short echo delays and caudal units to longer delays) is only observed at echo levels below 70 dB SPL or at higher echo levels when units are presented with long echo delays (that is, 20 and 22 ms). This ‘blurry’ activation pattern was also observed in the activation maps of individual P. parnellii and C. perspicillata (see Supplementary Figs S3 and S4 ). 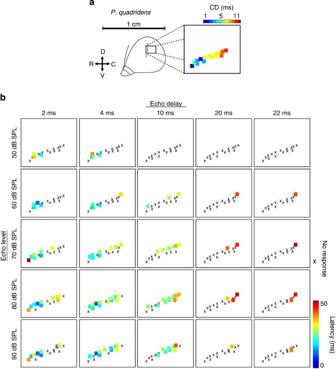Figure 6: Activation maps of oneP. quadridens. (a) Cortical distribution of CD. (b) Activation maps calculated for echo levels between 50 and 90 dB SPL and echo delays of 2, 4, 10, 20 and 22 ms. In the activation maps, units that fired below 50% of their maximum activity in response to a given echo delay–echo level combination (a situation considered as no response) were represented with an ‘x’. For the units that did respond to the echo delay–echo level combination, the latency of the response is represented in colours. Figure 6: Activation maps of one P. quadridens . ( a ) Cortical distribution of CD. ( b ) Activation maps calculated for echo levels between 50 and 90 dB SPL and echo delays of 2, 4, 10, 20 and 22 ms. In the activation maps, units that fired below 50% of their maximum activity in response to a given echo delay–echo level combination (a situation considered as no response) were represented with an ‘ x ’. For the units that did respond to the echo delay–echo level combination, the latency of the response is represented in colours. Full size image In the activation maps of Fig. 6b (and those in Supplementary Figs S3 and S4 ), the response latency of each unit at the specific echo delay is colour coded. A common observation in activation maps of all three species was that responses to longer delays had longer latencies than those to shorter delays. Longer latencies in response to longer echo delays were also observed in the dot raster plots that depict the response pattern of individual neurons ( Fig. 7 ). In all three species, delay-tuned neurons started to fire only after the presentation of the echo, and the latency of response unequivocally increased with the echo delay (see example neurons in Fig. 7 ). This timing result is in accordance with previous studies showing that pulse-evoked inhibition controls the latency of delay-tuned responses [25] . In all three species, the neuronal latency measured at the CD–MT point of the DRF was weakly correlated with the CD (that is, R =0.4 ( P. quadridens and P. parnellii ) and R =0.5 ( C. perspicillata ); see Supplementary Fig. S5 ). 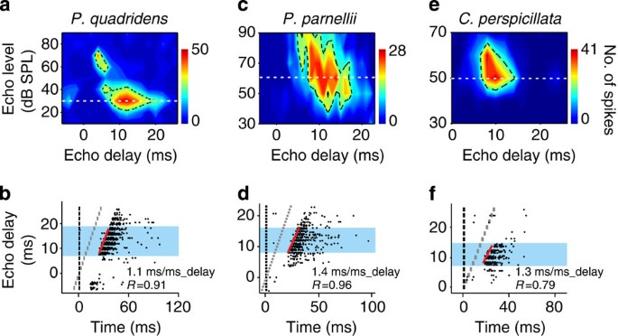Figure 7: Temporal response pattern of delay-tuned neurons. (a,b)P. quadridens, (c,d)P. parnelliiand (e,f)C. perspicillata. (a,c,e) DRFs of three units. The white dashed line indicates the unit’s BL. The example neuron fromP. quadridensand the one fromP. parnelliiwere tuned to heteroharmonic pulse–echo pairs in which the pulse mimicked the downward FM component of the fundamental biosonar harmonic (FM1), while the echo mimicked the second FM harmonic (FM2). The example neuron ofC. perspicillatawas tuned with homoharmonic combinations of the second harmonic (FM2). (b,d,f) Dot display of the response pattern of the same units at the BL. Black vertical lines indicate the temporal position of the pulse and grey vertical lines indicate the temporal position of the echo. Dots represent the spike times relative to the onset of the pulse. The regression line calculated with the response latencies at different echo delays is shown in red. The slope of the regression line and the correlation coefficient (R) are given. Response latency was calculated only for those stimulus pairs for which the response was above 50% of the maximum response (that is, those within the blue rectangles). Figure 7: Temporal response pattern of delay-tuned neurons. ( a , b ) P. quadridens , ( c , d ) P. parnellii and ( e , f ) C. perspicillata . ( a , c , e ) DRFs of three units. The white dashed line indicates the unit’s BL. The example neuron from P. quadridens and the one from P. parnellii were tuned to heteroharmonic pulse–echo pairs in which the pulse mimicked the downward FM component of the fundamental biosonar harmonic (FM1), while the echo mimicked the second FM harmonic (FM2). The example neuron of C. perspicillata was tuned with homoharmonic combinations of the second harmonic (FM2). ( b , d , f ) Dot display of the response pattern of the same units at the BL. Black vertical lines indicate the temporal position of the pulse and grey vertical lines indicate the temporal position of the echo. Dots represent the spike times relative to the onset of the pulse. The regression line calculated with the response latencies at different echo delays is shown in red. The slope of the regression line and the correlation coefficient ( R ) are given. Response latency was calculated only for those stimulus pairs for which the response was above 50% of the maximum response (that is, those within the blue rectangles). Full size image To characterize the relationship between echo delay and response latency at a population level, we calculated population latencies from all the neurons studied in each species. Populations latencies were calculated at an echo level of 70 dB SPL (because this echo level evoked a strong response in most delay-tuned neurons) and echo delays between 2 and 24 ms ( Fig. 8a ). Population latencies characterize the response of the group of neurons that respond to a specific echo delay regardless of whether it is its CD, BD, MinD or MaxD. Again, we observed that responses to longer echo delays had longer latencies than responses to shorter delays. In all three species, the median population latency of the subgroup of neurons that were responsive to the specific echo delays increased gradually with the studied echo delay, yielding correlation coefficients above 0.95 ( Fig. 8a ). 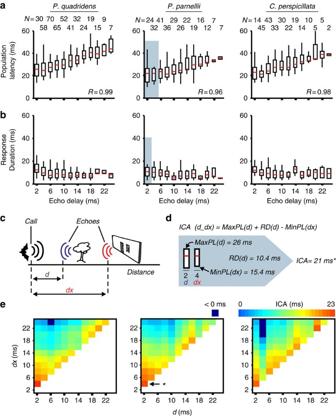Figure 8: Population response latencies and ICA. All measurements were made at an echo amplitude of 70 dB SPL. (a) Population latencies calculated in the three studied species at different echo delays. The number of neurons activated by a specific echo delay value is indicated above the graphs. In the boxplots, the upper border of each box was defined as MaxPL and the lower border was defined as MinPL. Horizontal lines inside the boxes indicate median population latencies and the whiskers extend to the most extreme data points not considered outliers. The linear correlation coefficient (R) calculated between the different echo delays and median population latencies is given. (b) Duration of responses to different echo delays. The median RD is represented by the horizontal line inside the boxes. (c) Schematic representation of a bat flying towards two objects with different space depths (that is, a tree and a wall), echo delays generated by each of the two objects are represented (that is,danddx). (d) Procedure for calculating the ICA for echo delays of 2 and 4 ms (danddx, respectively) inP. parnellii. The asterisk indicates the position of this ICA value in the ICA map calculated forP. parnellii(seee). (e) ICA maps that depict the time overlap of responses to different echo delays. Note that in all three species, responses to echo delays that are more similar are more likely to occur simultaneously in the cortex. Figure 8: Population response latencies and ICA. All measurements were made at an echo amplitude of 70 dB SPL. ( a ) Population latencies calculated in the three studied species at different echo delays. The number of neurons activated by a specific echo delay value is indicated above the graphs. In the boxplots, the upper border of each box was defined as MaxPL and the lower border was defined as MinPL. Horizontal lines inside the boxes indicate median population latencies and the whiskers extend to the most extreme data points not considered outliers. The linear correlation coefficient ( R ) calculated between the different echo delays and median population latencies is given. ( b ) Duration of responses to different echo delays. The median RD is represented by the horizontal line inside the boxes. ( c ) Schematic representation of a bat flying towards two objects with different space depths (that is, a tree and a wall), echo delays generated by each of the two objects are represented (that is, d and dx ). ( d ) Procedure for calculating the ICA for echo delays of 2 and 4 ms ( d and dx , respectively) in P. parnellii . The asterisk indicates the position of this ICA value in the ICA map calculated for P. parnellii (see e ). ( e ) ICA maps that depict the time overlap of responses to different echo delays. Note that in all three species, responses to echo delays that are more similar are more likely to occur simultaneously in the cortex. Full size image There was certain variability in the population latencies to the different echo delays. Such variability was quantified by measuring the quartiles (25th and 75th percentiles) of population latencies distributions (that is, represented by the boxes in Fig. 8a ). The 25th percentile (lower edge in the boxplots) is a measure of the minimum amount of time elapsed before the cortical FM/FM area is able to deliver a response to a given echo delay. This parameter was denoted as the minimum population latency (MinPL). On the other hand, the 75th percentile (upper edge in the boxplots) is a measure of maximum population latencies (MaxPLs). Together with the median response duration (RD) represented in Fig. 8b , MinPL and MaxPL provide an idea of the time window during which the FM/FM area holds activation in response to a certain echo delay. Intervals of concurrent activation (ICA) were calculated to determine the extent to which responses to different echo delays could occur simultaneously in the cortex. Bats have to deal with multiple echo delays produced from a single call emission whenever they fly towards objects with different space depths (a situation depicted in Fig. 8c ). Concurrent activations in response to different echo delays were hypothesized to be important for assembling complex acoustic images in E. fuscus [26] (a bat species that does not possess a topographically arranged target-distance map). ICAs were calculated according to the formula: ICA (d_dx) =MaxPL (d) +RD (d) − MinPL (dx) , where d indicates the value of a given echo delay and dx is any studied delay that is longer than d , MaxPL (d) and MinPL (dx) represent the minimum and maximum population latencies at d and dx , respectively, and RD (d) is the median RD calculated at d . Figure 8d exemplifies the procedure for calculating the ICA in P. parnellii for echo delays of 2 and 4 ms ( d and dx , respectively). The MaxPL calculated at 2 ms echo delay ( d , in this case) had a value of 26 ms and the median RD was 10.4 ms. The MinPL calculated for an echo delay of 4 ms ( dx , in this example) was 15.4 ms. These values yielded an ICA of 21 ms, which is the theoretical time window during which responses to delays of 2 and 4 ms could occur simultaneously in the FM/FM area of the mustached bat. In each species, ICAs were calculated for all possible d–dx combinations for echo delays between 2 and 24 ms, and they were colour-coded and plotted in the form of ICA maps ( Fig. 8e ). Our results indicate that in the cortex of P. quadridens , P. parnellii and C. perspicillata , long and short echo delays that indicate the presence of objects with different space depths can be concurrently represented by cortical neurons. However, the probability of binding objects together based on the timing of neuronal responses (probability as taken from ICA values) varies depending on the distance between the objects that are to be bound. In the ICA maps of all three species ( Fig. 8e ), for any given value of d , there was a gradual decrease in the ICA value as dx increased. The largest ICA values (dark red colours) were found in most cases towards the maps’ diagonal, indicating that the more similar two echo delays are (that is, the closer two targets are), the larger the probability that the responses they evoke coincide in time in the cortex. Target-distance maps are found in the FM/FM area of echolocating bats. The FM/FM area was proven to be instrumental for discriminating between echo delays during a fear conditioning task [8] . However, the mechanisms by which this area—and the map it contains—yields a representation of acoustic scenes during echolocation remains largely unknown. There are three main findings in the present study (i) the cortical target-distance maps appear differently depending on the bat species that is studied and the parameter of the delay receptive field that is used to construct these maps; (ii) the target-distance representation within the map is rather blurry, because the receptive field of adjacent neurons largely overlaps; and (iii) the bat species that possess a target-distance map also could profit from the timing of neuronal responses to build up complex acoustic images, as do bats that do not possess chronotopic maps [26] . From the three species studied here, C. perspicillata appears to have the most stable target-distance map across DRF metrics, followed by P. parnellii and P. quadridens (see Figs 3 and 4 ). It is unclear why these three species differ in the robustness of their cortical target-distance representations. What is clear from our data is that in the hunt for cortical topographies, experimenters should try to construct maps using several receptive-field parameters, and not just one. In the dorsal auditory cortex of bats, a topographic organization of delay-tuned neurons is more apparent for tuning measures that change more abruptly along the cortical surface (that is, CD and MaxD) and less apparent for measures that change at slower rates (that is MinD, see Fig. 5 and Supplementary Fig. S2 ). Measuring multiple receptive-field parameters also could yield more accurate interpretations about the functional roles of the auditory cortex. For example, the analysis of CD alone indicates that the FM/FM area of P. quadridens is best suited for the detection of rather distant targets, as the distribution of CDs is centred at 10 ms (1.7 m target distance). Such distribution could be of advantage for foraging in background cluttered environments [7] . However, the latter does not imply that delay-tuned neurons of P. quadridens are not well prepared for the detection of close targets, as the distributions of MinDs and BDs reveal that most units do respond to echo delays below 10 ms (see Fig. 2 ). Overall, the results from mapping multiple DRF metrics in the dorsal auditory cortex of bats confirm the thesis that the multiparametric nature of receptive fields obscures the appearance of cortical computational maps. The same has been shown for structural maps (that is, tonotopic maps that simply reproduce the peripheral representation of sensory information). The multiparametric nature of receptive fields is in the very essence of cortical function, although it might hamper our ability to measure maps. In bats, the multiparametric nature of receptive fields not only obscures the appearance of cortical target-distance maps but also adds a certain degree of blurriness to the map. For example, in the FM/FM area, most neurons respond (at least to some extent) to short echo delays and only a few respond to long delays (see Fig. 2 ). The few neurons that respond to long delays will be active when a distant object is detected, and this activation will be localized towards the caudal portion of the map (see Fig. 6 ). However, if the object is located in the immediate vicinity of the bat, then neurons throughout the map will respond and, therefore, activation within the map will not be precisely and unequivocally localized. Behavioural studies have shown that bats can discriminate between short target distances (that is, distances below 30 cm (~2 ms delay)) nearly without errors if the distances differ between them by at least 4 cm (0.2 ms delay) [27] . However, the activation pattern observed in the target-distance map suggests that when flying close to an object, there will be a low grain resolution that could lead into a decreased discrimination capability (based on the topology of cortical activation) but also into a categorical detection of short echo delays. The activation pattern of the cortical map cannot explain fine short-distance discriminations and, therefore, precise and unequivocally localized cortical activation might not be mandatory for a precise performance. Besides the bat, blurry maps for precise computations and/or behaviours have been found in the primary motor cortex that controls finger and wrist movements in primates [28] , the MT area of the visual cortex that encodes for direction of movement [29] and the map of sound-source localization in the owls’ tectum [18] . Perceptual issues aside, a stronger activation of the FM/FM area provides stronger output to other brain structures. The FM/FM area projects to other regions within the auditory cortex, but more importantly it has abundant projections to association areas such as the frontal cortex and to subcortical nuclei such as the auditory thalamus, inferior colliculi and the amygdala [30] . A stronger activation of the FM/FM area could be of advantage for fast initiation of motor responses required to resolve demanding situations such as prey catching or avoiding possible collisions. The latter is known as the ‘alarm hypothesis’ [5] . Our data also show that bats that possess chronotopic maps also could profit from the timing of neuronal responses for the analysis of complex scenes (see Fig. 8 ). Assembling acoustic images by binding cortical responses to different echo delays could work properly when echolocation calls are emitted at low repetition rates (that is, during the search phase of echolocation). Even in high duty cycle echolocators such as P. parnellii , during search flight, the interval between FM components of two consecutive biosonar calls is above 30 ms (see example search calls of P. parnellii in ref. 31 ). This interpulse interval is long enough to accommodate echoes from targets located as far as 5 m from each other, without any interference from echoes from the next emission. Avoiding overlaps between the streams of echoes generated from successive emissions seems to be important for bats, as they shift the frequency content of their calls if echoes from the first emission are still arriving at the time when a second call is produced [32] . Surgical and recording procedures The experiments were conducted on the left auditory cortex of 12 adult P. quadridens (7 females, 5 males), 10 adult P. parnellii (5 females, 5 males) and 9 adult C. perspicillata (5 females, 4 males). It was impossible to determine the exact age of the bats, but all of the studied animals were capable of sustained flight and echolocated actively. These two features have been observed only in adult bats or subadults when they reach the last developmental states [33] . Experiments on P. quadridens and P. parnellii were conducted in Cuba (Havana University) and experiments on C. perspicillata were conducted in Germany (Goethe University, Frankfurt am Main). P. parnellii and P. quadridens were captured in Cuban caves. Individuals of C. perspicillata were taken from a breeding colony at the Frankfurt University. All experiments comply with individual institutional guidelines and the Principles of Animal Care, Publication No. 86-23, revised 1985, of the National Institute of Health, and with the Declaration of Helsinki Principles. All experiments were conducted inside a sound-proof chamber. Bats were kept anaesthetized during the experiments. Different mixtures of anaesthetics were used in different species. P. quadridens was anaethesized with ketamine (10 mg kg −1 , Ketavet) and xylazine (20 mg kg −1 , Rompun). P. parnellii was anaesthetized with 10 mg kg −1 ketamine and 10 mg kg −1 pentobarbital (Sigma). C. perspicillata was anaesthetized with ketamine (10 mg kg −1 Ketavet) and xylazine (38 mg kg −1 Rompun). After anaesthesia, the muscles over the skull were carefully removed to expose the skull, and a hole was drilled to gain access to the FM/FM area. A carbon microelectrode (Carbostar-1, Kation Scientific, 0.4–0.8 MΩ) was used to record single and multi-unit activity. Cortical activity was amplified 10,000 times, filtered between 300 and 5,000 Hz using a differential extracellular amplifier (EX1 single-Channel Amplifier, Dagan Corporation) and finally digitized (sampling rate=31.3 kHz) and stored in a computer for offline analysis. Acoustic stimuli Acoustic stimuli were generated by a D/A board (DAP 840, Microstar Laboratories; sampling rate=278.8 kHz), attenuated (PA5, Tucker Davis Technologies), amplified (Avisoft Bioacoustics, Berlin, Germany; portable ultrasonic amplifier) and delivered from a calibrated speaker (ScanSpeak Revelator R2904/7000, Avisoft Bioacoustics). The speaker was placed at a distance of 15 cm, pointing in the direction of the bat’s right ear. The level of the presented stimuli was corrected online according to the calibration frequency response curve of the speaker. The calibration curve was obtained with a Brüel&Kjaer sound recording system (1/4-inch Microphone 4135, Microphone Preamplifier 2670) connected to a conditioning microphone amplifier (Nexus 2690). Pairs of FM sweeps mimicking call and echo were used to obtain DRFs. For the construction of DRFs, the temporal position and level of one of the artificial FM sweeps (defined as pulse) was held constant, whereas the temporal position and level of a second sweep (defined as echo) were randomly changed. Pulse level was set to 70 dB SPL for P. quadridens and P. parnellii and to 80 dB SPL for C. perspicillata . The frequency structure of pulse–echo pairs was adjusted so that it elicited the largest response of the delay-tuned neurons of each species. For example, P. quadridens and P. parnellii were presented with heteroharmonic pulse–echo pairs in which the fundamental downward FM component of the biosonar call (FM1: 41–28 kHz ( P. quadridens ) or 33–19 kHz) was followed with a certain delay by one of the higher FM harmonics (that is, FM2 or FM3 in P. quadridens and FM2, FM3 or FM4 in P. parnellii ). In C. perspicillata , delay tuning was studied using homoharmonic pulse–echo pairs. For homoharmonic stimulation, pairs of sounds with similar spectral composition that mimicked either the second (FM2: 45–93 kHz) or third biosonar harmonics (FM3: 70–125 kHz) were presented with a certain delay. Characterization of DRFs Responses were analysed offline using custom-made Matlab scripts. Recorded spikes were discriminated using a spike-sorting procedure based on the three principal components of the spike waveforms and the posterior use of a software for unsupervised classification of multidimensional data (that is, KlustaKwik [34] , [35] ). Only the largest cluster of waveforms was selected for subsequent analysis. In spite of the efforts made to isolate responses from single units, contributions of more than one unit to the studied response cannot be ruled out. DRFs were visualized as filled contour plots ( contourf function, Matlab). Threshold curves were calculated as 50% of the maximum response in the DRF. The DRF of each neuron was characterized by measuring the MT and CD (that is, the delay and echo level at the lowest tip of the threshold curve); BD and BL (that is, the delay and echo level that evoked the unit’s maximum response); and MinD and MaxD calculated in the threshold curves at the MinD level and MaxD level, respectively. Post-stimulus time histograms (PSTHs) of responses to the different echo delay–echo level combinations were constructed with a bin width of 1 ms. RD was measured as the 50% width in the PSTHs. Response latencies were measured from the onset of the FM sweep defined as pulse to the time at which the neuronal response reached 50% of the maximum of the PSTHs at the rising slope of the histogram. Construction of cortical maps Coordinates of each neuron in the cortical surface were measured during the experiments using the ocular scale of the surgical microscope (20 μm resolution at × 50 magnification, Carl Zeiss Stemi 2000c). In all three species, the rostrocaudal position of neurons was determined relative to a large branch of the median cerebral artery that overlaid the Sylvian sulcus. This physical coordinate was then normalized in each animal relative to the position of the most rostral neuron that had a CD of 2 ms. In P. quadridens and C. perspicillata , the dorsoventral coordinate was taken relative to the lower edge of the pseudocentral sulcus. In P. parnellii , the dorsoventral coordinate was taken relative to the more ventral edge of the physiological FM1/FM4 border, that is, the more ventral neuron that was tuned to a combination of FM1 (pulse) and FM4 (echo), and not to FM1/FM2 or FM1/FM3. Cortices from different animals were aligned together for the construction of composite maps. The Sylvian sulcus and median cerebral artery were used as references to determine the orientation of the ordinate axis in the bidimensional Cartesian space of analysis. A gradient analysis was conducted to determine the spatial orientation of composite maps. The gradient of a function of two variables (that is, F(x, y) , where F is the response property of interest (that is, the CD) and x and y indicate coordinates of each recording site) is expressed as a collection of vectors pointing in the direction of increasing values of F . Gradient vectors were calculated in each individual animal and their angular orientation was accumulated and plotted in the form of circular scatter plots. Two parameters were used for characterization of circular scatter plots, that is, the mean angular direction ( α ) and mean vector magnitude ( L α ). The value of α indicates the angular orientation of a particular circular distribution. L α is a measure of the distribution variance ( V ), it is calculated by the formula L α =1 −V . Rayleigh’s test was used to further measure circular uniformity. In Rayleigh’s test, a P <0.05 indicates an angle distribution that is not circularly uniform. All circular statistics were computed using the CircStat toolbox designed for Matlab [36] . Activation maps Activation maps were calculated for each animal. These maps do not depict the distribution of DRF parameters along the cortical surface but rather provide a visual representation of the neurons that are activated by a given echo delay–echo level combination. A unit was arbitrarily defined to respond to a given echo delay–echo level combination whenever the combination evoked a response larger than 50% of the unit’s maximum response to all tested echo delay–echo level combinations. In the activation maps, the latency of responses was measured and colour coded for visual representation. How to cite this article: Hechavarría, J. C. et al . Blurry topography for precise target-distance computations in the auditory cortex of echolocating bats. Nat. Commun. 4:2587 doi: 10.1038/ncomms3587 (2013).